Defective Hfp-dependent transcriptional repression ofdMYCis fundamental to tissue overgrowth inDrosophilaXPB models Nucleotide excision DNA repair (NER) pathway mutations cause neurodegenerative and progeroid disorders (xeroderma pigmentosum (XP), Cockayne syndrome (CS) and trichothiodystrophy (TTD)), which are inexplicably associated with (XP) or without (CS/TTD) cancer. Moreover, cancer progression occurs in certain patients, but not others, with similar C-terminal mutations in the XPB helicase subunit of transcription and NER factor TFIIH. Mechanisms driving overproliferation and, therefore, cancer associated with XPB mutations are currently unknown. Here using Drosophila models, we provide evidence that C-terminally truncated Hay/XPB alleles enhance overgrowth dependent on reduced abundance of RNA recognition motif protein Hfp/FIR, which transcriptionally represses the MYC oncogene homologue, dMYC . The data demonstrate that dMYC repression and dMYC-dependent overgrowth in the Hfp hypomorph is further impaired in the C-terminal Hay/XPB mutant background. Thus, we predict defective transcriptional repression of MYC by the Hfp orthologue, FIR, might provide one mechanism for cancer progression in XP/CS. For cell cycle patterning of multicellular animals, cells must have the capacity to quickly respond to extracellular developmental signals. Recent work has highlighted the importance of poised (transcriptionally engaged, but paused) RNA Polymerase II (RNA Pol II) on the promoters of Drosophila embryonic patterning genes as a mechanism to facilitate rapid and synchronous transcription in response to secreted morphogens [1] , [2] , [3] , [4] , [5] , [6] , [7] . Preceding this interest in RNA Pol II pausing, earlier ex vivo studies identified poised RNA Pol II at the transcriptional start site (TSS) of the MYC oncogene [8] , [9] , [10] . MYC drives cell growth and cell cycle progression [3] , [11] and is frequently dysregulated in cancer [12] , [13] , [14] , [15] . dMYC is the sole MYC family member in Drosophila [16] , [17] , [18] and is functionally homologous to MYC [16] , [19] , [20] , [21] , [22] . As even subtle increases in MYC expression (more than twofold) can promote cancer initiation and progression, MYC abundance must be tightly regulated [14] , [15] , [16] , [23] , [24] . Due to the short half life and low steady-state abundance of both MYC mRNA and protein, multiple mechanisms operate to constrain MYC (for example, transcription, mRNA turnover, translation and protein degradation) [16] , [23] , [25] , [26] , [27] , [28] , [29] , [30] , [31] , [32] . Ex vivo studies suggest paused, but transcriptionally engaged, RNA Pol II at the start site of the MYC promoter provides (1) rapid response to mitogenic signals and (2) protection from unwanted promoter activation [16] , [33] , [34] . Activation of RNA Pol II is dependent on general transcription factor IIH (TFIIH) [35] , [36] , a multi-subunit complex essential for nucleotide excision repair (NER) and RNA Pol II-dependent transcription [7] , [16] , [23] , [24] . The complex genetic disorders xeroderma pigmentosum (XP), Cockayne syndrome (CS), trichothiodystrophy (TTD) and combined XP/CS are caused by mutations in NER genes, including XPB (encoded by ERCC3 ) the helicase subunit of TFIIH [16] , [24] , [37] , [38] , [39] . In contrast to CS and TTD, which are not associated with cancer, XP patients are extremely photosensitive and have a 1,000-fold increased risk of skin cancer, and 10-to-20 times higher risk of internal cancers [1] , [3] , [5] , [7] , [40] . However, despite years of study investigating the NER pathway in this group of diseases the outstanding question remains—why do certain mutations result in cancer phenotypes in some patients, but not others? Although >28 NER proteins have been implicated in XP, TTD, CS and XP/CS, other than XPB, only the XPD helicase and TTDA are TFIIH subunits. TTDA is required for the stability of the TFIIH complex, but unlike XPB and XPD, which are implicated in all three diseases, defects in TTDA only cause the developmental disease TTD, not XP/CS and/or cancer [8] , [41] . Intriguingly, three different XPB families with mutations in ERCC3 , the gene coding XPB, causing loss of the wild-type C terminus of XPB, all display the severe neurodegenerative progeroid disorder characteristic of CS, but have different cancer predisposition (one severe, one moderate, one with no cancer) [3] , [41] , [42] . Altogether with the knowledge that all patients in these families have reduced NER, these observations suggest that cancer phenotypes are not due to NER defects per se , but likely due to a second mutation. Thus we predict that XPB-dependent DNA repair defects are not the direct cause of cancer phenotypes, but are a consequence of additional hyperproliferative input(s), perhaps involving the transcription of a gene driving tissue overgrowth. Serum stimulation of mammalian tissue culture cells results in a rapid increase in MYC transcription [12] , [43] , which is associated with release of RNA Pol II from the TSS [16] , [44] . Subsequently, RNA Pol II is restored to the TSS and MYC transcription is returned to basal levels, consistent with the poised RNA Pol II complex at the MYC TSS being required to shut down MYC [16] , [43] . Indeed at other gene promoters, paused RNA Pol II appears to govern inappropriate transcription, presumably as a consequence of steric hindrance from the multi-subunit RNA Pol II complex blocking stochastic recruitment of RNA Pol II [20] , [22] , [44] . XPB regulates post-initiation control of MYC transcription via the RNA recognition motif protein FIR and the KH domain protein FBP [16] , [23] , [24] , [45] . Specifically, under the conditions of activated (serum stimulated) MYC transcription, XPB is required for recruiting both FBP and FIR to a single-stranded promoter sequence (the far upstream sequence element) 1.7 kB upstream of the MYC TSS [16] , [23] , [40] . FIR is recruited subsequent to the peak in MYC , is proposed to inactivate RNA Pol II and is required to return MYC transcription to basal levels [16] , [41] . Indeed, loss-of-function FIR mutations are associated with colorectal cancer with increased MYC abundance [3] , [35] . Thus, proper control of MYC transcription likely requires physical interaction between FIR and XPB [16] , [23] , [24] , [43] . However, it is unclear whether post-initiation control via RNA Pol II pausing in the MYC promoter is required for in vivo control of MYC transcription. Intriguingly, ex vivo studies suggest physical interaction between FIR and XPB lacking the wild-type C terminus are defective in cells from one patient with severe XP/CS and multiple cancers (XP11BE) [16] , [24] , [38] , [40] , but whether other XPB patient mutations affect the interaction with FIR is unknown. Given the role in controlling abundance of the MYC oncogene, we hypothesized that altered interactions between XPB and FIR may contribute, at least in part, to malignancy in patients with XPB mutations. Haywire (Hay) is the Drosophila XPB homologue [40] , [41] , [43] , [44] , and loss-of-function Hay mutants display increased cell death, consistent with DNA repair and/or transcription defects [41] , [42] , [46] . The Drosophila orthologue of FIR, Half Pint (Hfp) behaves as a tumour suppressor, as loss of Hfp results in larval overgrowth and overproliferation [43] , [44] . Hay forms a complex with Hfp in vivo and co-ablation of Hay in Hfp loss-of-function cells reduces dMYC expression and cell growth [44] , [47] , [48] , [49] . Altogether these data suggest conservation between mammalian FIR-XPB and Drosophila Hfp-Hay in terms of transcriptional regulation of MYC and growth control. Here we demonstrate that C-terminally truncated Hay mutants enhance the larval overgrowth associated with reduced Hfp abundance [18] , [43] , [50] , [51] . Moreover, we show that animal overgrowth depends on elevated dMYC, thus providing further support for the homology between Hfp and FIR in regards to their capacity to repress MYC transcription via XPB/Hay [44] , [52] , [53] . Altogether, these data suggest mutations disrupting FIR function have the potential to promote XPB-related cancers. Hay mutants modify Hfp-dependent overgrowth The alignment between the Human XPB -mutation associated with XP/CS disease and the Hay mutations used here are shown in Fig. 1a . The conserved domains between the Human-XPB and Drosophila -Hay protein are highlighted and include the N-terminal DNA binding domain, several helicase domains and the C-terminal domain. The Drosophila Hay nc2 allele was first identified in 1988 [45] , [54] and characterized as a point mutation at amino-acid position 652 in the sixth helicase domain [18] , [40] , [50] , [51] , [54] . Subsequently, following ethyl methane sulfonate-induced mutagenesis, several other Hay mutants were generated in the Hay nc2 background and molecularly characterized [41] , [54] . The original Hay nc2 point mutation affects the conserved helicase domain but encodes an in-frame C-terminal domain, whereas the ethyl methane sulfonate mutants chosen for analysis here ( Hay nc2rv1 , Hay nc2rv3 , Hay nc2rv7 ) contain stop codons at position 657, 380 and 441, respectively, and lack the C-terminal domain ( Fig. 1a ). These mutants have been selected because mutations of XPB encoding a C-terminally truncated protein have been implicated in XP/CS [3] , [55] ( Fig. 1a ). 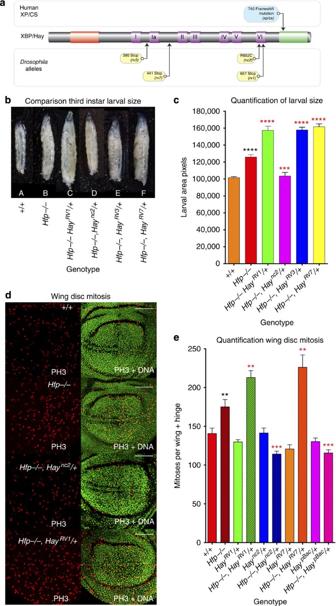Figure 1:Haymutants differentially modify overgrowth and proliferation of hypomorphicHfpmutants. (a) Alignment ofXPBandHayshowing mutations associated with XP/CS compared withDrosophilamutant alleles. Conserved domains include; N terminal (red), helicase (purple) and Carboxy-terminal (green). (b)Haymutant alleles differentially modify the third instar larval overgrowth phenotype for theHfphypomorph. (c) quantified larval area (seeSupplementary Table 1for quantification and number of biological replicates). (d)Haymutant alleles differentially modify overproliferation ofHfphypomorphs. Third instar larval wing imaginal discs stained with anti-phosphohistone H3 (PH3). All scale bars represent 50 μm. (e) quantification of mitosis (seeSupplementary Table 2for quantification and biological replicates). The black asterisks show significance points compared with control; red asterisks compared withHfphypomorph alone. Statistical tests for this figure and all following figures were performed with Graphpad Prism 6 using unpaired two-tailedt-test with 95% confidence interval. In all figures error bars represent s.e.m. and according to the Graphpad classification of significance points *P=0.01 to 0.05, **P=0.001–0.01, ***P=0.0001–0.001 and ****P<0.0001. Figure 1: Hay mutants differentially modify overgrowth and proliferation of hypomorphic Hfp mutants. ( a ) Alignment of XPB and Hay showing mutations associated with XP/CS compared with Drosophila mutant alleles. Conserved domains include; N terminal (red), helicase (purple) and Carboxy-terminal (green). ( b ) Hay mutant alleles differentially modify the third instar larval overgrowth phenotype for the Hfp hypomorph. ( c ) quantified larval area (see Supplementary Table 1 for quantification and number of biological replicates). ( d ) Hay mutant alleles differentially modify overproliferation of Hfp hypomorphs. Third instar larval wing imaginal discs stained with anti-phosphohistone H3 (PH3). All scale bars represent 50 μm. 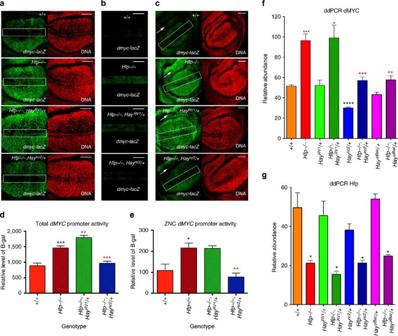Figure 2:Haymutants differentially modifydMYC-promoter activity associated with theHfphypomorph. (a)dMYC–lacZactivity detected with anti β-gal (green) and DAPI (red) for genotypes marked. The rectangles mark the D-V boundary. (b)dMYC-lacZacross the D/V boundary. (c) lower magnification view to showdMYC–lacZin the hinge (marked with a white arrow in the dorsal region). All scale bars represent 50 μm. (d) Quantification ofdMYC–lacZactivity across the wing disc and (e) across the D/V boundary. The graphs in D and E show the relative intensity for β-gal antibody staining (mean β-gal pixel intensity±s.e.m.) for each genotype (Supplementary Table 3for quantification and number of biological replicates). (f-g) ddPCR fordMYCandHfpmRNA abundance in wing discs, normalized to tubulin (seeSupplementary Table 4for quantification and number of biological replicates). The black asterisks show significance points compared with control; red asterisks compared withHfphypomorph alone. Statistical tests were performed with Graphpad Prism 6 using unpaired two-tailedt-test with 95% confidence interval. In all figures error bars represent s.e.m. and according to the Graphpad classification of significance points *P=0.01–0.05, **P=0.001–0.01, ***P=0.0001–0.001 and ****P<0.0001. ( e ) quantification of mitosis (see Supplementary Table 2 for quantification and biological replicates). The black asterisks show significance points compared with control; red asterisks compared with Hfp hypomorph alone. Statistical tests for this figure and all following figures were performed with Graphpad Prism 6 using unpaired two-tailed t -test with 95% confidence interval. In all figures error bars represent s.e.m. and according to the Graphpad classification of significance points * P =0.01 to 0.05, ** P =0.001–0.01, *** P =0.0001–0.001 and **** P <0.0001. Full size image The Hfp EP contains an enhancer P element insertion in the 5′-UTR of Hfp , 94 bp upstream of the initiating methionine and expresses reduced Hfp ( Fig. 2 ) [43] , [56] . Homozygous Hfp EP larvae and pupae are ∼ 20% larger than wild-type third instar larvae, due to increased proliferation during the third larval instar ( Fig. 1b–e ). Homozygosity for the Hay mutant alleles is embryonic lethal, consistent with the helicase function being essential for transcription and DNA repair [40] , [55] . Although heterozygosity for the Hay alleles alone does not result in overproliferation ( Fig. 1d,e and discussed below), we observed that one copy of particular Hay alleles modified the larval overgrowth phenotype associated with the hypomorphic Hfp mutant ( Fig. 1b,c , P <0.0001, Supplementary Table 1 ) [18] , [43] , [57] , [58] . The Hay nc2 allele significantly suppressed ( Fig. 1b,c , P =0.0004) and, conversely, Hay nc2rv1 significantly enhanced ( Fig. 1b,c , P <0.0001), the Hfp larval overgrowth phenotype. Similarly, two additional Hay alleles ( Hay nc2rv3 and Hay nc2rv7 ) lacking the C-terminal domain, and 5–6 of the helicase domains (that is, this deletion also removes the original point mutation at amino-acid position 652 in the sixth helicase domain), significantly enhanced the Hfp overgrowth phenotype ( Fig. 1b,c , P <0.0001, Supplementary Table 1 ). Figure 2: Hay mutants differentially modify dMYC- promoter activity associated with the Hfp hypomorph. ( a ) dMYC – lacZ activity detected with anti β-gal (green) and DAPI (red) for genotypes marked. The rectangles mark the D-V boundary. ( b ) dMYC-lacZ across the D/V boundary. ( c ) lower magnification view to show dMYC – lacZ in the hinge (marked with a white arrow in the dorsal region). All scale bars represent 50 μm. ( d ) Quantification of dMYC – lacZ activity across the wing disc and ( e ) across the D/V boundary. The graphs in D and E show the relative intensity for β-gal antibody staining (mean β-gal pixel intensity±s.e.m.) 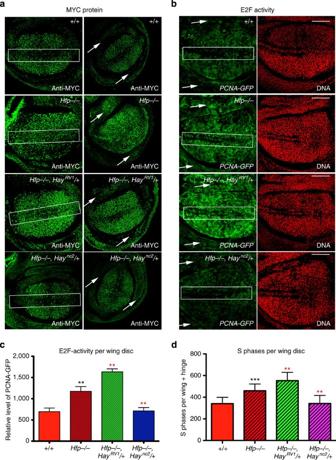Figure 3:Haymutants differentially modify MYC protein patterning, E2F-activity and S phase progression inHfphypomorphs. (a) MYC antibody staining (green) for genotypes marked. The white rectangles mark the ZNC and white arrows mark the hinge domain. All scale bars represent 50 um. (b) PCNA–GFP activity (green) and DAPI (red) for genotypes marked. (c) Quantification ofPCNA–GFPactivity. The graph shows the relative intensity for GFP (mean pixel intensity±s.e.m.) for each genotype (seeSupplementary Table 5for quantification and number of biological replicates). (d) Quantification of S phase using BrdU. The graph shows number of BrdU positive cells (±s.e.m.) in wing discs for genotypes marked (seeSupplementary Table 6for quantification and number of biological replicates). The black asterisks show significance points compared with control; red asterisks compared withHfphypomorph alone. Statistical tests were performed with Graphpad Prism 6 using unpaired two-tailedt-test with 95% confidence interval. In all figures error bars represent s.e.m. and according to the Graphpad classification of significance points *P=0.01–0.05, **P=0.001–0.01, ***P=0.0001–0.001 and ****P<0.0001. for each genotype ( Supplementary Table 3 for quantification and number of biological replicates). 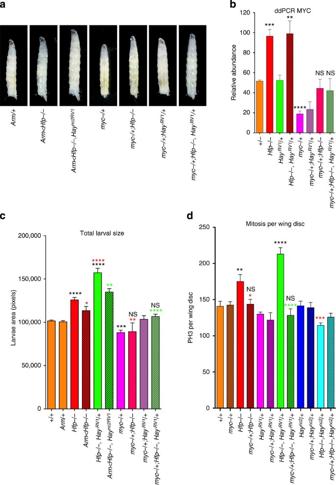Figure 4: Larval overgrowth and proliferation is dependent on dMYC. (a) Light microscope images of third instar larvae for genotypes marked. (b) ddPCR fordMYCandHfpmRNA abundance in wing discs, normalized to tubulin (seeSupplementary Table 9for quantification and number of biological replicates). (c) Quantification of larval area. The graph shows the mean pixel area (±s.e.m., seeSupplementary Table 8for quantification and number of biological replicates). (d) Quantification of mitosis per wing disc for the genotypes marked. The graph shows the mean PH3 count (±s.e.m.; seeSupplementary Table 10for quantification and number of biological replicates). The black asterisks show significance points compared with control; red asterisks compared withHfphypomorph alone and green asterisks compared withHaync2RV1in theHfphypomorph background. Statistical tests were performed with Graphpad Prism 6 using unpaired two-tailedt-test with 95% confidence interval. In all figures error bars represent s.e.m. and according to the Graphpad classification of significance points *P=0.01–0.05, **P=0.001–0.01, ***P=0.0001–0.001 and ****P<0.0001. ( f-g ) ddPCR for dMYC and Hfp mRNA abundance in wing discs, normalized to tubulin (see Supplementary Table 4 for quantification and number of biological replicates). The black asterisks show significance points compared with control; red asterisks compared with Hfp hypomorph alone. Statistical tests were performed with Graphpad Prism 6 using unpaired two-tailed t -test with 95% confidence interval. In all figures error bars represent s.e.m. and according to the Graphpad classification of significance points * P =0.01–0.05, ** P =0.001–0.01, *** P =0.0001–0.001 and **** P <0.0001. Full size image Suppression of growth by the Hay nc2 point mutant is consistent with our observation that reduced Hay abundance suppressed overgrowth from loss of Hfp [18] , [44] , [57] . However the Hay alleles lacking the C-terminal domain behave counter to what would be predicted for loss-of-function Hay mutations, which suggests the C-terminal domain may be required for growth repression. To characterize the counter-intuitive observation that the C-terminally truncated Hay mutants ( Hay nc2rv1 , Hay nc2rv3 and Hay nc2rv7 ) enhance the Hfp phenotype we next analysed cell cycle markers in the larval wing imaginal discs from these animals. Hay mutants modify cell division in the Hfp hypomorph To determine whether the larval overgrowth ( Fig. 1b,c ) was associated with increased proliferation we measured mitosis in larval wing imaginal discs. Hypomorphic Hfp discs had significantly more PH3 cells, compared with wild type ( Fig. 1d,e , P =0.0084, Supplementary Table 2 ) and, in line with the observation that heterozygous Hay mutants do not overgrow, levels of mitosis were not significantly altered by the point mutant or C-terminally truncated Hay alleles alone ( Fig. 1e ). The Hay allele with the smallest C-terminal truncation ( Hay nc2RV1 ) significantly increased mitosis compared with the Hfp hypomorph alone ( Fig. 1d,e , P =0.0073). Thus, Hay nc2RV1 can only promote overproliferation in the context of reduced Hfp. Similarly, the Hay nc2RV7 mutant, which lacks the C-terminal domain including the point mutation at position 652, did not result in overproliferation alone, but significantly increased mitosis in the Hfp hypomorph background ( Fig. 1e , P =0.0082). In contrast, the point mutant ( Hay nc2 ) significantly decreased PH3 compared with the Hfp hypomorph alone, to return mitosis to the wild type range ( Fig. 1d,e , Supplementary Table 2 , P =0.0002). Similarly, heterozygosity for Hay loss-of-function mutations generated by P-element insertion in the Hay open-reading frame ( PBac{WH}hayf00028 ), which will lead to reduced abundance of wild type protein [46] , [59] , significantly decreased mitosis compared with Hfp alone ( Fig. 1e , P =0.001). Altogether these data suggest repression of cell cycle by Hfp [44] , [60] , [61] , is sensitive to the level and function of Hay. However, since increased proliferation was not observed for the C-terminal truncated mutants alone, this suggests the C-terminal domain of Hay is only required for repression of cell cycle when Hfp is reduced. Thus we next investigated whether increased growth and proliferation was associated with changes to dMYC transcription. dMYC transcription in Hfp mutants is sensitive to Hay The wing imaginal disc is an epithelial sheet, which can be subdivided into notum, hinge and wing pouch regions, based on the fate of each of these structures in the adult. Developmental signalling events set up compartment boundaries within the wing disc to define anterior–posterior (A/P) and dorsoventral (D/V) compartments [47] , [48] , [49] , [62] . In particular, dMYC expression is downregulated across the D/V boundary to form the presumptive wing margin during the third larval instar and, as a consequence, cells are delayed in the cell cycle and form a ‘zone of non-proliferating cells’ (ZNC) at the D/V boundary [18] , [50] , [51] , [62] ( Fig. 2a ). To investigate changes to dMYC transcription we used a dMYC-lacZ enhancer trap, which reflects dMYC promoter activity. B-gal was detected in the cycling cells of the third instar wing pouch and reduced both along the differentiating cells at the D/V boundary and throughout the hinge domain [52] , [53] , [57] ( Fig. 2a,c ), consistent with patterning of dMYC mRNA [54] , [62] . dMYC enhancer trap activity spanning the entire wing disc (pouch and hinge) was significantly greater in Hfp mutants compared with wild type ( Fig. 2a,c , quantified in 2D, P =0.0003, Supplementary Table 3 ) and further significant increases were observed in the Hay nc2rv1 background ( Fig. 2a,c quantified in 2D, P =0.0052). Conversely, the Hay point mutant reduced dMYC promoter activity in the Hfp hypomorph ( Fig. 2a,c , quantified in 2D P =0.0003). Altogether, these data suggest modulation of growth and proliferation in the Hfp hypomorph by the Hay alleles is due, at least in part, to differential effects on dMYC promoter activity. As highlighted above, dMYC is downregulated along the D/V boundary of the wing disc in preparation for cell cycle exit and differentiation of sensory bristles along the adult wing margin (rectangles in Fig. 2a,c ) [16] , [18] , [23] , [24] , [50] , [51] , [54] . dMYC mRNA is detected in the second instar hinge, which forms circular domains that surround the pouch, but is normally downregulated in third instar [44] , [54] , as reflected by the pattern of dMYC enhancer trap activity ( Fig. 2c , white arrow). Ectopic dMYC-lacZ activity was observed along the D/V boundary and within the presumptive hinge of Hfp hypomorphs ( Fig. 2a–c ). Significantly higher levels of promoter activity were detected throughout the D/V boundary of Hfp mutants compared with the control ( Fig. 2b,e , P =0.0319). Although dMYC-lacZ was still detected throughout the ZNC for Hfp mutants in the presence of the C-terminally deleted Hay nc2rv1 allele, a further increase in dMYC promoter activity was not observed across the wing margin ( Fig. 2b,e ). The Hay point mutant significantly reduced dMYC-lacZ activity compared with the Hfp mutant alone ( Fig. 2b,e , P =0.0035, Supplementary Table 3 ), such that dMYC promoter activity was not significantly different from wild type. We also observed continued dMYC promoter activity in the hinge of the Hfp mutant wing discs ( Fig. 2c , white arrow). Suppression of dMYC-lacZ activity in the hinge was observed for the Hay point mutant compared with Hfp mutant alone, however, enhancement by the C-terminally truncated mutant was difficult to ascertain as the β-gal signal was already saturated in the Hfp mutant background ( Fig. 2c , arrows). Broadly, however, Hfp mutants alone significantly increased dMYC promoter activity, which was further increased by the C-terminally truncated Hay protein and, conversely, suppressed by the Hay point mutant. To determine whether altered dMYC promoter activity was associated with changes to productive transcription we quantified dMYC mRNA abundance in third instar wing imaginal discs using digital PCR (with probes spanning the 3′ exon-intron boundary of the most 3′ exon). As expected Hfp mRNA was significantly decreased in the hypomorphic background ( Fig. 2g , P >0.05 for the Hfp hypomorph alone and in the Hay nc2RV1 , Hay nc2 and Hay pBac backgrounds compared with wild type, see Supplementary Table 4 ). Importantly, we found a significant increase in dMYC mRNA in the Hfp hypomorph compared with the wild-type control ( Fig. 2f , P =0.0005). dMYC mRNA was also significantly increased in hypomorphic Hfp wings heterozygous for Hay nc2RV1 ( Fig. 2f , P =0.0101 compared with wild type, see Supplementary Table 4 ). The increased proliferation observed in the Hay nc2rv1 background was not, however, associated with a further increase in dMYC mRNA abundance. This could be a consequence of negative feedback loops, whereby increased dMYC abundance leads to autorepression at the level of transcription [55] , [63] . Specifically, and consistent with the autorepression first suggested for mammalian MYC [56] , [64] , overexpression of dMYC reduces endogenous dMYC transcription [55] . Thus, although there is a similar twofold increase in dMYC at this stage of wing development, an earlier increase in dMYC activity associated with Hay nc2rv1 may have induced a program of enhanced proliferation. Importantly, heterozygosity for the Hay point mutant or P-element mutant significantly decreased dMYC mRNA compared with the Hfp hypomorph alone ( Fig. 2f Hay nc2 P =0.006 and Hay pBac , P =0.0059, Supplementary Table 4 ). Indeed dMYC mRNA levels in Hfp hypomorphs heterozygous for Hay nc2 or Hay pBac were not significantly different from wild type. dMYC antibody staining of wing discs revealed that disrupted patterning of the dMYC promoter was associated with altered dMYC protein localization. As predicted hypomorphic Hfp wings from 3rd instar larvae had an overall increase in dMYC antibody staining, particularly in the ZNC and hinge ( Fig. 3a ). Heterozygosity for the C-terminal Hay mutant in the Hfp hypomorph further increased dMYC abundance, particularly the ectopic dMYC in the hinge and across the D/V boundary. As anticipated, given the decrease in proliferation in wing discs for Hfp mutants heterozygous for the Hay point mutant, dMYC protein was decreased, and this was particularly clear in the hinge ( Fig. 3a ). To determine whether the altered dMYC promoter activity, mRNA and protein abundance was associated with changes to dMYC function we next monitored S phase progression in wing discs. Figure 3: Hay mutants differentially modify MYC protein patterning, E2F-activity and S phase progression in Hfp hypomorphs. ( a ) MYC antibody staining (green) for genotypes marked. The white rectangles mark the ZNC and white arrows mark the hinge domain. All scale bars represent 50 um. ( b ) PCNA–GFP activity (green) and DAPI (red) for genotypes marked. ( c ) Quantification of PCNA – GFP activity. The graph shows the relative intensity for GFP (mean pixel intensity±s.e.m.) 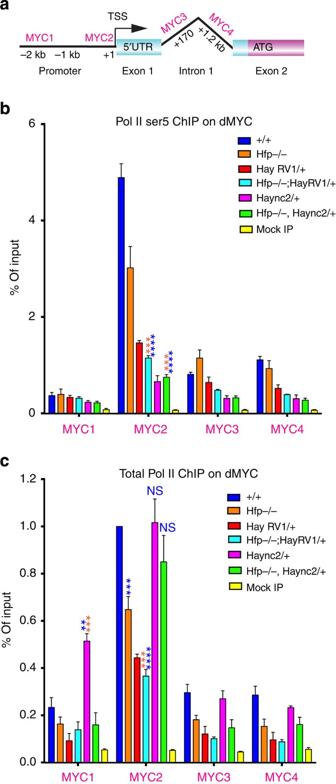Figure 5:Haymutants affect RNA Pol II enrichment across thedMYCpromoter. (a) Schematic ofdMYCshowing the position of the amplicons used for qPCR. (b) ChIP for Ser 5 RNA Pol II and (c) ChIP for total RNA Pol II (seeSupplementary Table 11,12for quantification and number of biological replicates). Statistical tests were performed with Graphpad Prism 6 using unpaired two-tailedt-test with 95% confidence interval. In all figures error bars represent s.e.m. and according to the Graphpad classification of significance points *P=0.01–0.05, **P=0.001–0.01, ***P=0.0001–0.001 and ****P<0.0001. for each genotype (see Supplementary Table 5 for quantification and number of biological replicates). ( d ) Quantification of S phase using BrdU. The graph shows number of BrdU positive cells (±s.e.m.) in wing discs for genotypes marked (see Supplementary Table 6 for quantification and number of biological replicates). The black asterisks show significance points compared with control; red asterisks compared with Hfp hypomorph alone. Statistical tests were performed with Graphpad Prism 6 using unpaired two-tailed t -test with 95% confidence interval. In all figures error bars represent s.e.m. and according to the Graphpad classification of significance points * P =0.01–0.05, ** P =0.001–0.01, *** P =0.0001–0.001 and **** P <0.0001. Full size image S phase activity in Hfp mutants is sensitive to Hay dMYC drives cell growth and couples this with progression through the cell cycle via activation of S phase genes [18] , [57] , [58] . In particular, dMYC promotes initiation of DNA synthesis/S phase via upregulation of the G1-S cyclins, Cyclin E and Cyclin D [18] , [57] , which pair with the Cyclin-dependent kinases (CDKs), Cdk2 (ref. 59 ) and Cdk4 (refs 60 , 61 ), respectively. The Cyclin/CDK complexes can phosphorylate and inactivate the Retinoblastoma protein (Rb) homologue Rbf to release the E2F transcription factor to activate expression of the S phase genes [62] . A key target of E2F and its binding partner DP is the DNA replication factor, proliferating cell nuclear antigen (PCNA) [62] . Increased dMYC activity will, therefore, lead to upregulation of E2F1 function [57] , which can be measured using a PCNA–GFP reporter [62] . The PCNA–GFP pattern in wing discs shows E2F activity throughout dividing cells in the wing pouch and the expected decrease across the D/V boundary in wild-type discs ( Fig. 3b ). In line with the abnormal pattering of the dMYC enhancer trap, increased dMYC mRNA ( Fig. 2 ) and protein ( Fig. 3a ), ectopic PCNA–GFP activity was observed across the presumptive wing margin and throughout the hinge of Hfp mutant discs ( Fig. 3b , Supplementary Figure 1 ) and GFP intensity was significantly greater in the Hfp hypomorph compared with wild type ( Fig. 3c , P =0.009, see Supplementary Table 5 ). In accordance with the C-terminally truncated Hay allele further increasing dMYC activity, PCNA–GFP activity was significantly increased across the wing pouch, compared with the Hfp mutant alone ( P =0.0028, Fig. 3c ). Conversely, the Hay point mutant significantly decreased E2F-activity in the Hfp mutant background ( P =0.0070, Fig. 3c ). Moreover, the Hay nc2 point mutant reduced PCNA–GFP activity across the ZNC ( Fig. 3b ) and the hinge ( Supplementary Figure 1 ). The increased PCNA–GFP activity was also associated with cell cycle progression; BrdU incorporation revealed that Hfp mutants had significantly more cells in S phase than control ( Fig. 3d , P =0.0004, see Supplementary Table 6 ). S phases were further increased by the Hay nc2RV1 C-terminal deletion and reduced by the Hay nc2 point mutant ( Fig. 3d , P =0.0077 and P =0.0022, respectively). Thus the C-terminally truncated Hay protein further increases dMYC -promoter activity and S phase progression, suggesting increased dMYC-activity drives the overproliferation and larval overgrowth and wing disc overproliferation in the Hfp mutant background ( Fig. 1 ). dMYC is critical for Hfp and Hay dependent overgrowth We next demonstrated that the overgrowth associated with Hay nc2RV1 was dependent on reduced Hfp and/or elevated dMYC. As shown above, Hfp mutants alone, or in the heterozygous Hay nc2RV1 background, were significantly larger than wild type ( Fig. 1b,c , P <0.0001 for both). Ubiquitous overexpression of Hfp from the enhancer P, which is inserted in the Hfp promoter and contains UAS sites, with the Arm-GAL4 driver ( Supplementary Table 7 and Supplementary Figure 2 for quantification of Hfp and MYC mRNA) resulted in significantly reduced overgrowth of hypomorphic Hfp larvae, both alone and in the Hay nc2RV1 background ( Fig. 4a,c , P =0.0331 and P =0.0318 compared with Hfp alone, Supplementary Table 8 ). Thus, overgrowth in these animals was dependent on decreased abundance of Hfp. Figure 4: Larval overgrowth and proliferation is dependent on dMYC. ( a ) Light microscope images of third instar larvae for genotypes marked. ( b ) ddPCR for dMYC and Hfp mRNA abundance in wing discs, normalized to tubulin (see Supplementary Table 9 for quantification and number of biological replicates). ( c ) Quantification of larval area. The graph shows the mean pixel area (±s.e.m., see Supplementary Table 8 for quantification and number of biological replicates). ( d ) Quantification of mitosis per wing disc for the genotypes marked. The graph shows the mean PH3 count (±s.e.m. ; see Supplementary Table 10 for quantification and number of biological replicates). The black asterisks show significance points compared with control; red asterisks compared with Hfp hypomorph alone and green asterisks compared with Hay nc2RV1 in the Hfp hypomorph background. Statistical tests were performed with Graphpad Prism 6 using unpaired two-tailed t -test with 95% confidence interval. In all figures error bars represent s.e.m. and according to the Graphpad classification of significance points * P =0.01–0.05, ** P =0.001–0.01, *** P =0.0001–0.001 and **** P <0.0001. Full size image Importantly, overgrowth of Hfp hypomorphs, either alone or in the Hay nc2RV1 background, was dependent on elevated dMYC. Specifically, heterozygosity for the dMYC mutant ( dm P0 ), which returned dMYC mRNA levels to the wild-type range in wing imaginal discs ( Fig. 4b ; Supplementary Table 9 ), significantly decreased larval growth ( Fig. 4a,c P =0.025 for Hfp −/− and P <0.0001 Hfp−/−, Hay nc2RV1 , Supplementary Table 8 ). Mitosis was also returned to the wild-type range in wing imaginal discs heterozygous for an alternate dMYC mutant ( dm G0354 ; Fig. 4c , P =0.0132 for Hfp −/− and P <0.0001 for Hfp −/− , Hay nc2RV1 Supplementary Table 10 ). Altogether these data suggest that the increased animal overgrowth and overproliferation in the Hfp hypomorph, and further growth driven by Hay nc2RV1 , is dependent on elevated dMYC. Hay mutants differentially alter RNA Pol II pausing on dMYC Control of mammalian MYC transcription requires interaction between the Hfp (FIR) and Hay (XPB) orthologues ex vivo [16] , [23] , [24] , thus, we hypothesized that the Hay-Hfp interaction [44] might regulate transcription in vivo via RNA Pol II activity within the dMYC promoter. We therefore used ChIP to monitor RNA Pol II enrichment across the dMYC promoter, using antibodies specific to the C-terminal domain (CTD) of the largest RNA Pol II subunit ( Fig. 5 ). RNA Pol II is recruited to gene promoters in a hypophosphorylated (inactive) state and promoter escape requires TFIIH-mediated phosphorylation of the Ser5 residue of the CTD of the largest subunit [63] . Thus antibodies specific to (1) the Ser-5 phosphorylated isoform and (2) all isoforms of the CTD were used for ChIP. Figure 5: Hay mutants affect RNA Pol II enrichment across the dMYC promoter. ( a ) Schematic of dMYC showing the position of the amplicons used for qPCR. ( b ) ChIP for Ser 5 RNA Pol II and ( c ) ChIP for total RNA Pol II (see Supplementary Table 11,12 for quantification and number of biological replicates). Statistical tests were performed with Graphpad Prism 6 using unpaired two-tailed t -test with 95% confidence interval. In all figures error bars represent s.e.m. and according to the Graphpad classification of significance points * P =0.01–0.05, ** P =0.001–0.01, *** P =0.0001–0.001 and **** P <0.0001. Full size image ChIP from wild-type imaginal discs revealed a peak of RNA Pol II (Ser5 and total) proximal to the dMYC transcriptional start site ( Fig. 5b,c , blue columns), which suggests dMYC transcription is regulated by RNA Pol II pausing in vivo . The RNA Pol II detected using the total RNA Pol II antibody is therefore likely to be predominantly Ser5 phosphorylated, suggesting most of the RNA Pol II on dMYC is normally poised for promoter escape and transcription. In contrast to control, the Hfp hypomorph had significantly decreased Ser5 and total RNA Pol II enrichment across the dMYC TSS ( Fig. 5b , P =0.0052, Fig. 5c , P =0.0007, respectively Supplementary Tables 11,12 ). This suggested reduced levels of Hfp, which are associated with increased dMYC expression, impair RNA Pol II pausing across the dMYC promoter. Thus we investigated whether the Hay mutants might differentially affect RNA Pol II to account for the altered dMYC promoter activity/transcription ( Fig. 2 ). Interestingly, the Hay nc2RV1 C-terminal deletion further decreased enrichment for both Ser5 and RNA Pol II ( Fig. 5b , P <0.0001) and total RNA Pol II ( Fig. 5c , P =0.0018) in the Hfp hypomorphic background (that is, compared with Hfp alone), suggesting a further reduction in RNA Pol II pausing might explain the increased dMYC activity ( Fig. 2 ). However, the observation that there is less Ser 5 RNA Pol II and total RNA Pol II on the dMYC promoter for the Hay nc2RV1 C-terminal mutant alone, but no increase in dMYC expression or cell growth, suggests that the decrease in paused RNA Pol II alone is not sufficient to hyperactivate dMYC . Rather, heterozygosity for the C-terminal truncation sensitizes dMYC to further hyperactivation when Hfp levels are reduced. Altogether this suggests that Hfp levels are key to the hyperactivation of dMYC transcription, as reduced RNA Pol II pausing alone is not sufficient for dMYC promoter activation when Hfp is abundant. Although the Hay nc2 point mutant was also associated with a further decrease in Ser5 RNA Pol II enrichment across the TSS in both the wild type and the Hfp mutant background ( Fig. 5b , P <0.0001 for both Hay nc2 and Hfp −/− , Hay nc2 compared with control), enrichment for total RNA Pol II was in the control range ( Fig. 5c ). Together this suggests nonphosphorylated and, therefore, inactive/paused RNA Pol II holoenzyme accumulates on the dMYC TSS in the Hay nc2 background. Thus, although RNA Pol II loading occurs in these mutants, the fraction of Ser5 phosphorylated isoform appears to be reduced relative to holoenzyme, which would be expected to reduce RNA Pol II pause release from the dMYC promoter and impair transcription (that is, as observed in Fig. 2 ). The significant reduction in dMYC expression in the Hay nc2 mutants compared with reduced Hay abundance, which does not alter dMYC mRNA levels (that is, using the Hay pBac mutant, Fig. 2f ), might be explained by the initial molecular characterization demonstrating the Hay nc2 allele encodes a stable protein, that is much more abundant than the wild-type Hay protein [41] . Hay nc2 might, therefore, be expected to not only impair TFIIH activity, but to also block activity of the wild type protein. Thus we predict the Hay nc2 mutant inhibits precocious release of RNA Pol II and activation of dMYC normally associated with reduced Hfp repressor, as non-functional, stable protein blocks wild type Hay function. Together these data provide an explanation for how the Hay alleles differentially modify dMYC-dependent overgrowth in the Hfp hypomorph; (1) being enhanced by the Hay nc2RV1 C-terminal deletion due to further impairment of dMYC repression and (2) being suppressed by the Hay nc2 point mutant due to increased accumulation of inactive RNA Pol II on the dMYC promoter. The XPB helicase is a multi-function protein, being required to unwind DNA before all RNA Pol II-dependent transcription [64] , and for both transcription-coupled repair and global genome repair of DNA damage [2] , [4] , [6] , [65] . The complex disease phenotypes in XP/CS families are emphasized by patients carrying C-terminal mutations in XPB , who have combined Xeroderma pigmentosum/Cockayne syndrome (XP/CS), with or without cancer [3] , [9] , [10] . In vivo mouse models carrying the C-terminal XPB mutation have failed to elucidate clear mechanisms underlying cancer phenotypes in XPB-related diseases. XPB/XPCS knockin mice developed to mimic XPB-related XP/CS, by encoding a C-terminally truncated protein, are indistinguishable from wild-type animals. Intriguingly, challenging the DNA repair pathways by placing the XPB/XPCS heterozygotes in an NER-deficient background (double mutant for the Xpa repair protein) did not significantly increase spontaneous tumour incidence [11] , [66] . Thus mammalian studies have left unresolved the question of why mutations in the C-terminal domain of XPB result in cancer in some patients, but not others. On the basis of our Drosophila models, we predict that malignancies observed in cancer prone XP/CS families (III and IV) [3] , [13] , [14] , [15] might be due to mutations affecting FIR abundance, which we would expect to promote MYC-dependent overproliferation in the context of the XPB C-terminal mutation. In contrast we would predict that the XP/CS family V, which has not shown cancer phenotypes [3] , [17] , [18] , has normal FIR abundance/function. Interestingly of the other TFIIH components associated with TTD, XP, CS or XP/CS, the XPD helicase is implicated in all three diseases, including XP with increased ultraviolet-induced cancer incidence, while the TTDA protein has only been linked to the developmental disease TTD. In the repair pathway, the XP-related NER endonucleases (XPG and XPF) also only have increased cancer incidence in response to ultraviolet-irradiation. Our observations from Drosophila suggest that the increased propensity of XPB patients with the C-terminal truncation to cancer might be due to specific roles for XPB in mediating Hfp/FIR-dependent repression of MYC transcription. The Drosophila models demonstrate that like the heterozygous XPB/XPCS knockin mice, Hay nc2RV1 heterozygotes do not overproliferate, but enhance cell and tissue overgrowth in a manner dependent on reduced abundance of the dMYC repressor, Hfp. The interaction between Hay and Hfp is of particular interest as, like Hay/XPB, Hfp has been implicated as a dual function protein. Initially, due to the presence of the RNA recognition motif it was implicated in RNA splicing in Drosophila [19] , [67] . However, our work suggests Hfp also behaves as a dMYC transcriptional repressor, likely via binding single-stranded DNA to maintain RNA Pol II pausing on the dMYC promoter. In mammals, FIR splice variant mutations lacking exon 2, which encodes the transcriptional repression domain, are associated with colorectal cancer and are hypothesized to promote tumour development by disrupting FIR-dependent MYC repression [28] . In accordance with dMYC being the core target in flies, we demonstrate overgrowth in the Hfp hypomorph, either alone or in the C-terminally truncated Hay background, is associated with defective repression of dMYC promoter activity and dependent on elevated dMYC. The diminished enrichment of RNA Pol II across the dMYC TSS, both in the Hfp hypomorph alone, and exacerbated by the Hay C-terminal truncation, suggests the interaction between Hay and the Hfp-repressor might be required for maximal RNA Pol II pausing. This is supported by the observations that in cells from an XP/CS patient with severe and multiple cancers (XP11BE), where the XPB protein lacks the wild-type C terminus; (1) MYC transcription is dysregulated, (2) the direct interaction (via GST pull-down assays) normally observed between XPB and FIR is not detected for XPB protein and (3) FIR enrichment on MYC is maintained at the far upstream sequence element, but decreased at the promoter, suggesting impaired promoter looping [16] , [21] , [23] , [24] . Consistent with this, the Hay nc2RV1 C-terminal mutant significantly decreases RNA Pol II enrichment on the dMYC promoter compared with the Hfp hypomorph alone ( Fig. 5 ), and is associated with increased dMYC promoter activity, and dMYC-dependent animal growth and proliferation ( Figs 1 , 2 , 3 , 4 ). The notion that paused RNA Pol II can behave as an insulator to suppress inappropriate transcription from paused promoters [14] , [15] , [20] , [22] is supported by the enhancement of dMYC expression and overgrowth correlating with a further reduction in RNA Pol II enrichment on the dMYC promoter. Moreover, accumulation of nonphosphorylated RNA Pol II across the dMYC promoter in the Hay nc2 background is associated with decreased dMYC transcription, both alone and in the Hfp mutant background. Hfp-dependent transcriptional mechanisms, therefore, underlie the role of Hay in controlling dMYC abundance and animal growth in vivo . In particular, the interaction between Hay and Hfp is required to maintain RNA Pol II pausing, which we predict will normally block inappropriate transcription from the dMYC promoter. Altogether the data suggest that dysregulated transcriptional repression of MYC by the human Hfp orthologue, FIR, in addition to defective DNA repair, might also contribute to cancer progression in XPB-related human diseases. These predictions are consistent with human ex vivo experiments suggesting physical interaction between FIR, the Hfp orthologue and MYC repressor, and XPB is defective in cell lines derived from a cancer prone XP/CS patient with the C-terminal XPB mutation [16] , [24] , [25] , [26] , [27] , [28] , [29] , [30] , [31] , [32] . Our observation that a single copy of the C-terminally truncated XPB homologue, Hay, increases abundance of dMYC and cell cycle progression in Hfp hypomorphs suggests that loss of this MYC -repressor confers susceptibility to overgrowth in vivo . Specifically, the data suggest that impaired RNA Pol II pausing and precocious RNA Pol II release in the Hfp mutant background is exacerbated by the C-terminal Hay mutant, to result in further dMYC transcription and overproliferation. Finally, our findings suggest the interaction between Drosophila Hay/Hfp and mammalian XPB/FIR is likely conserved and, therefore, that loss-of-function FIR mutations might dictate whether certain XP patients are more likely to develop neoplastic malignancies. Fly strains Unless otherwise stated, the Drosophila strains were obtained from the Bloomington Stock Centre. PBac{WH}hayf00028 was from the Genomic mapping of Exelixis insertion collection [33] , [34] , [46] . The dMYC RNAi line (v2948) was obtained from the Vienna Drosophila RNAi Center [36] , [68] . PCNA–GFP was a gift from R. Duronio. Immunohistochemistry Larval imaginal tissues were fixed for 30 min in 4% PFA, blocked in 5% BSA in PBST at room temperature for 1 h before incubation overnight at 4 °C with the primary antibody and detection with fluorescently tagged secondary antibody. Primary antibodies included; β-gal (Sigma) (1:500); pH3 (millipore, 1:1,000), BrdU (Becton Dickinson, 1:100), dMYC (Santa Cruz (1/200) and anti-GFP (to detect PCNA-GFP only, Invitrogen). After counter-staining with DAPI and placing in 80% glycerol, wing imaginal discs were dissected and imaged with the Zeiss Imager Z confocal microscope using Zen Meta software. Z-series with 0.5 μm sections were performed at 40 × magnification. Fluorophores were imaged using band-pass filters to remove cross-detection between channels. Images were processed and prepared using Image J 1.43 μ, and Adobe Photoshop CS6 Version 11.0.2. Pixel intensity for PCNA-GFP and dMYC-lacZ activity was calculated using ImageJ from 3 × 0.5 μm confocal Z stacks (each genotype imaged at the same pinhole and gain) from the surface of the wing imaginal disc epithelium. Mitoses were quantified by measuring the ratio of average phosphohistone H3-positive cells per fixed area in the PC compared to the AC over at least 7 discs. Statistical tests were performed with Graphpad Prism 6 using unpaired 2-tailed t-test with 95% confidence interval. Bromodeoxyuridine labelling Larval imaginal tissues were incubated for 30 min in 100 μg ml −1 BrdU in Schneider’s media with 10% FCS followed by fixation in 4% PFA. Tissues were incubated in PBST at 37 °C for 30 min followed by DNAse treatment at 37 °C for 1.5 h and immunostained as described above with primary antibody for BrdU (Becton Dickinson, 1:100). Ratio of average BrdU-positive cells per fixed area in the PC compared with AC was calculated over at least seven discs. Statistical tests were performed with Prism 6 using unpaired two-tailed t -test with 95% confidence interval. cDNA synthesis and Droplet Digital PCR Third instar wing discs (10 pairs per genotype) were collected, RNA was extracted (Promega ReliaPrep RNA Cell Miniprep system) and eluted in 30 μl nuclease-free water. RNA purity and integrity was assessed using an automated electrophoresis system (2200 TapeStation, Agilent Technologies). Six microlitres of the eluted RNA samples were used for cDNA synthesis (Bioline Tetro cDNA Synthesis kit). For each genotype ddPCR (Droplet Digital PCR) was carried out on biological triplicates and quantified using the QX100 Droplet Digital PCR system (Bio-Rad) following the Digital MIQE guidelines [7] , [69] . The ddPCR mix consisted of: 10 μl 2 × ddPCR™ super mix for probes (Bio-Rad); 500 nM of primers for MYC and HFP, 250 nM of probe mix for MYC and HFP (Integrated DNA Technologies) and 1 μl of cDNA into a final volume of 20 μl. The total mix was placed into the eight-channel cartridge, 70 μl of droplet generating oil was added and droplets were formed in the QX100droplet generator (Bio-Rad). Droplets in oil suspensions were transferred to a 96 well plate and placed into the C1000 Touch™ Thermal Cycler (Bio-Rad). Cycling conditions were as follows: 95 °C for 10 min, followed by 40 cycles of 94 °C for 30 sec and 60 °C for 60 s. The droplets were subsequently read automatically by the QX100 droplet reader (Bio-Rad) and the data were analysed with the QuantaSoftsoftware 1.3.2.0 (Bio-Rad). The primers used were; MYC—5′-GTGGACGATGGTCCCAATTT-3′ 3′-GGGATTTGTGGG TAGCTTCTT-5′; HFP—5′-CCAGCATGAATCTCTTTGATTTGG-3′ 3′-GGAGTTCGTTGTGGGACAG-5′ The probes used were; MYC – 5′-/56-FAM/CCCTCAGAT/ZEN/TCCGATGAGGAAATCGA/3IABkFQ/-3′ and HFP—5′-/5HEX/TCGATCTAT/ZEN/TACGCCGCCGAATGC/3IABkFQ/-3′ Chromatin Immunoprecipitation ChIP assays were carried out as described with modifications [37] , [39] , [70] . For each ChIP sample, 30 larval heads were fixed in 4% paraformaldehyde for 20 min. Larval heads were then mashed and chromatin sheared in 0.4% SDS using a Covaris S2 (10 min duration, 10% DUTY, 200 cycles per burst, Intensity 4, achieving average DNA fragment sizes 200–600 bp). ChIPs were performed in IP buffer containing 0.1% SDS and 3 μg of antibody was used for each IP (anti-RNA Polymerase II phospho S5 antibody (ab5131) or Total RNA Polymerase CTD repeat 8WG16 (ab817, Abcam). Analysis was performed in triplicate using SYBR green dye (Bioline) on the ABI Prism 7900ht (Applied Biosystems). To calculate the percentage of total DNA bound, non-immuno precipitated input samples from each condition were used as reference for all qPCR reactions. The primers for qPCR were; MYC1—5′-GGCGATCGTTTCTGGCCTACGG-3′ 3′-GCAGGCGCATTTGACTCGGC-5′; MYC2—5′-TTTCTACCATGCGGCCTAAC-3′ 3′-GCTTTGGCGCCTTACATTTC-5′ MYC3—5′-ACTACTACTAACAACTGTCACAAGCCAAGT-3′ 3′-TTTATGTATTTGCGCGGTTTTAAG-5′; MYC4—5′-TTCAAAATAGAATTTCTGGGAAAGGT-3′ 3′ GCGGCCATGATCACTGATT 5′ MYC5—5′-GGTTTTCCTTTTATGCCCTTG-3′ 3′-CTATTAACCATTTGAACCCGAAATC-5′. How to cite this article : Lee, J.E.A. et al. Defective Hfp-dependent transcriptional repression of dMYC is fundamental to tissue overgrowth in Drosophila XPB models. Nat. Commun. 6:7404 doi: 10.1038/ncomms8404 (2015).